Epigenetic analysis leads to identification ofHNF1Bas a subtype-specific susceptibility gene for ovarian cancer HNF1B is overexpressed in clear cell epithelial ovarian cancer, and we observed epigenetic silencing in serous epithelial ovarian cancer, leading us to hypothesize that variation in this gene differentially associates with epithelial ovarian cancer risk according to histological subtype. Here we comprehensively map variation in HNF1B with respect to epithelial ovarian cancer risk and analyse DNA methylation and expression profiles across histological subtypes. Different single-nucleotide polymorphisms associate with invasive serous (rs7405776 odds ratio (OR)=1.13, P =3.1 × 10 −10 ) and clear cell (rs11651755 OR=0.77, P =1.6 × 10 −8 ) epithelial ovarian cancer. Risk alleles for the serous subtype associate with higher HNF1B -promoter methylation in these tumours. Unmethylated, expressed HNF1B , primarily present in clear cell tumours, coincides with a CpG island methylator phenotype affecting numerous other promoters throughout the genome. Different variants in HNF1B associate with risk of serous and clear cell epithelial ovarian cancer; DNA methylation and expression patterns are also notably distinct between these subtypes. These findings underscore distinct mechanisms driving different epithelial ovarian cancer histological subtypes. Invasive epithelial ovarian cancer (EOC) has a strong heritable component [1] , with an approximate three-fold increased risk associated with a first-degree family history [2] . Much of the excess familial risk observed for EOC is unexplained [3] , and efforts to identify common susceptibility genes have proven to be difficult. Seven regions harbouring susceptibility single-nucleotide polymorphisms (SNPs) for ovarian cancer have been identified through genome-wide association studies [4] , [5] , [6] , [7] thus far, but candidate gene studies have been largely unsuccessful [8] . The Cancer Genome Atlas (TCGA) has fully characterized more than 500 serous EOC cases with respect to somatic mutation, DNA methylation, mRNA expression and germline genetic variants [9] . These data are publicly available and can be analysed to identify candidate genes for association studies of the disease. We conducted such an analysis of TCGA data and found a unique expression and methylation pattern of HNF1B characterized by downregulation of expression in most cases, with epigenetic silencing in about half of the cases, suggesting it might have a role in the serous subtype of ovarian cancer. In contrast, HNF1B overexpression is common in clear cell ovarian cancer [10] . The HNF1B gene (formerly known as TCF2 ) encodes a POU-domain containing a tissue-specific transcription factor, and mutations in the gene cause maturity onset diabetes of the young type 5 (ref. 11 ). HNF1B is also a susceptibility gene for type II diabetes [12] , [13] , prostate cancer [12] , [14] , [15] , [16] and uterine cancer [17] . We report here on our comprehensive characterization of this gene in ovarian cancer and show evidence of a differential effect of HNF1B on the serous and clear cell subtypes of ovarian cancer. It appears that HNF1B has a loss-of-function role in serous and a gain-of-function role in clear cell ovarian cancers, and variants in this gene differentially affect genetic susceptibility to these subtypes. DNA methylation/expression analysis From TCGA data (see Methods ), HNF1B was observed to be epigenetically silenced in approximately half of the 576 primary serous ovarian tumours and downregulated by another mechanism in most of the other tumours, whereas no evidence of methylation was seen in the normal fallopian tube samples ( Fig. 1a , Supplementary Fig. S1 ) available from TCGA. We further assessed HNF1B -promoter methylation in an independent data set (OCRF panel; see Methods ) and found the promoter region to be methylated in 42% of serous tumours and in none of the clear cell ovarian tumours ( Fig. 1b ). The pattern in serous tumours, in contrast to clear cell cancers, led to the evaluation of HNF1B as a candidate subtype-specific susceptibility gene for ovarian cancer. 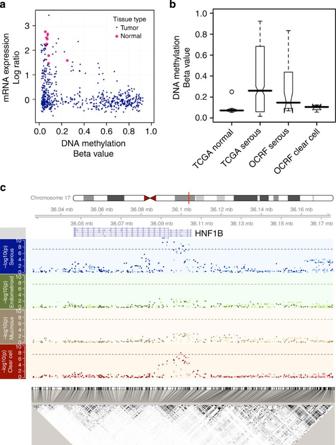Figure 1: Identification ofHNF1Bas a subtype-specific candidate gene for ovarian cancer and its establishment as a susceptibility gene. (a) The scatterplot compares the mRNA expression (y axis) versus DNA methylation (x axis) in serous ovarian tumours from TCGA (seeMethods). Each blue dot is a serous tumour sample, whereas each pink dot is one of the ten normal fallopian tube samples. TheHNF1Bpromoter is silenced in the majority of these tumours, either by an epigenetic (bottom right, high DNA methylation and low mRNA expression) or an unknown alternative mechanism. The mRNA expression data were integrated from three platforms (onlineMethods) and interpreted as log ratios, and we observe the same pattern with each individual expression platform (Supplementary Fig. S1). (b)HNF1B-promoter DNA methylation differs by histological subtype. Although unmethylated in the normal fallopian tissue, this locus is hypermethylated (beta value >0.2) in approximately 50% of the TCGA (n=576; seeMethods) serous cases as well as another independent set of 32 serous tumour samples (OCRF panel; seeMethods), but remains unmethylated in clear cell tumours (OCRF panel; seeMethods) (n=4). These data are consistent with reported HNF1B expression in the clear cell tumours. (c) Genetic variants in the HNF1B locus are associated with risk of ovarian cancer histological subtypes. Plotted in each panel is the −log10 (P-value) from the SNP association with risk for each subtype (Manhattan plots) located in the 150-kb region described in the text. Imputed SNPs are indicated with a relatively lighter colour, whereas the genotyped SNPs are indicated with a darker colour. Dashed lines indicate the genome-wide significance threshold (5 × 10−8). The linkage disequilibrium plot on the bottom shows ther2between the SNPs. Genomic coordinates are based on hg19 (Build37). Figure 1: Identification of HNF1B as a subtype-specific candidate gene for ovarian cancer and its establishment as a susceptibility gene. ( a ) The scatterplot compares the mRNA expression (y axis) versus DNA methylation (x axis) in serous ovarian tumours from TCGA (see Methods ). Each blue dot is a serous tumour sample, whereas each pink dot is one of the ten normal fallopian tube samples. The HNF1B promoter is silenced in the majority of these tumours, either by an epigenetic (bottom right, high DNA methylation and low mRNA expression) or an unknown alternative mechanism. The mRNA expression data were integrated from three platforms (online Methods ) and interpreted as log ratios, and we observe the same pattern with each individual expression platform ( Supplementary Fig. S1 ). ( b ) HNF1B -promoter DNA methylation differs by histological subtype. Although unmethylated in the normal fallopian tissue, this locus is hypermethylated (beta value >0.2) in approximately 50% of the TCGA ( n =576; see Methods ) serous cases as well as another independent set of 32 serous tumour samples (OCRF panel; see Methods ), but remains unmethylated in clear cell tumours (OCRF panel; see Methods ) ( n =4). These data are consistent with reported HNF1B expression in the clear cell tumours. ( c ) Genetic variants in the HNF1B locus are associated with risk of ovarian cancer histological subtypes. Plotted in each panel is the −log10 ( P -value) from the SNP association with risk for each subtype (Manhattan plots) located in the 150-kb region described in the text. Imputed SNPs are indicated with a relatively lighter colour, whereas the genotyped SNPs are indicated with a darker colour. Dashed lines indicate the genome-wide significance threshold (5 × 10 −8 ). The linkage disequilibrium plot on the bottom shows the r 2 between the SNPs. Genomic coordinates are based on hg19 (Build37). Full size image SNP analysis With all invasive cancer subtypes considered together, we found no genome-wide significant ( P <5 × 10 −8 ) HNF1B SNP associations among women of European ancestry ( Table 1 ; Supplementary Data S1 ). However, when analyses were stratified by histological subtype, we observed genome-wide significant results for both serous and clear cell EOC subtypes, but with risk associations in opposite directions. The association was similar for high- and low-grade serous cancers. There was no evidence of association for mucinous or endometrioid subtypes ( Fig. 1c ). Associations in the non-European populations are shown in Supplementary Table S2 . Table 1 Association between invasive, serous and clear cell ovarian cancer for ten HNF1B SNPs that reached genome-wide significance in Whites. Full size table Minor alleles at nine SNPs, six genotyped and three imputed, were associated with increased risk of invasive serous ovarian cancer at P <5 × 10 −8 ( Table 1 ). The risk signal spanned a 21.4-kb region from the 5′ untranslated region (UTR) through part of intron 4 of HNF1B ( Fig. 1c ). The most strongly associated SNP for invasive serous ovarian cancer (rs7405776, minor allele frequency (MAF) 36%) conferred a 13% increased risk per minor allele ( P =3.1 × 10 −10 ; Table 1 , Supplementary Fig. S2A ). The signals of this SNP and the eight other genome-wide significant SNPs were indistinguishable, given the linkage disequilibrium and resulting haplotype structure ( Supplementary Figs S3, S4 and S5 ). For the clear cell subtype, rs11651755 (MAF 45%) was associated with a 23% decreased risk of disease at a genome-wide significant level ( P =2 × 10 −8 ; Table 1 , Supplementary Fig. S2B ). This signal was distinct from the nine significant SNPs for invasive serous cancer ( Table 1 ). The odds against the serous-associated SNP, rs7405776, as the true best hit for clear cell ovarian cancer were 244:1. Conversely, the odds against the clear cell SNP, rs11651755, as the true best hit for serous were 1808:1. Further, when rs11651755 and rs7405776 were jointly modelled, the signal for clear cell cancer was driven completely by rs11651755, whereas that for the serous disease was driven by rs7405776 ( Table 1 ). The clear cell SNP (rs11651755) sits on five haplotypes, only three of which also contain the serous SNP (rs7405776; Supplementary Fig. S5 ). Thus, different SNPs in the HNF1B gene regions explain the associations observed for serous and clear cell ovarian cancer. DNA methylation and protein expression The identification of HNF1B as a susceptibility gene for serous and clear cell ovarian cancer led us to further evaluate the relationship between HNF1B -promoter DNA methylation, protein expression and histological subtype. Immunohistochemistry (IHC) analysis for HNF1B protein expression in 1,149 ovarian cancers from the Ovarian Tumor Tissue Analysis Consortium, and DNA-methylation analysis on 269 of these tumours, revealed that the majority of clear cell tumours expressed the HNF1B protein and were unmethylated at the HNF1B promoter, whereas the majority of serous tumours lacked HNF1B protein expression and displayed frequent HNF1B -promoter methylation ( Fig. 2 , Supplementary Fig. S6 ). 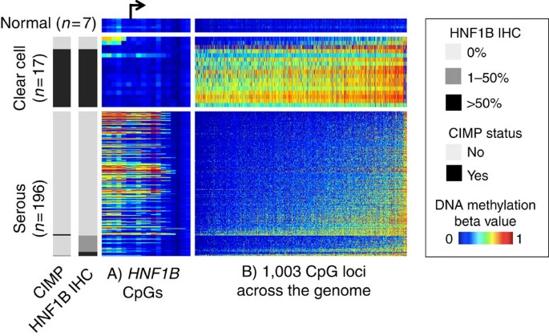Figure 2:HNF1B-promoter DNA methylation, protein expression and global DNA-methylation pattern by subtype. Each row is a tissue sample collected at the Mayo Clinic that belongs to one of the three categories: normal ovarian tissue (n=7), clear cell ovarian tumours (n=17) or serous ovarian tumours (n=196). Endometrioid (n=49) and mucinous (n=7) tumours are not included in this figure. Each column represents a CpG locus, either from the region flanking the HNF1B transcription start site (panel A, ordered by genomic locations with an arrow indicating the transcription start site) or from a global panel of 1,003 CpG loci mapped to autosomal CpG island regions that distinguish clear cell and serous subtypes (panel B, ordered by average DNA methylation across the samples). For each horizontal panel group, the samples (rows) are ordered by HNF1B IHC status. The heatmap shows the DNA-methylation beta value, with blue indicating low DNA methylation and red indicating high methylation. Clear cell tumours showed less DNA methylation at theHNF1B-promoter region and correspondingly higher HNF1B protein expression. The clear cell tumours generally show a CIMP where there is extensive gain of aberrant promoter methylation in a correlated manner. CIMP status (left side bar, defined as methylated at >80% of the 1,003 loci) is highly correlated HNF1B expression. Also noteworthy is that theHNF1B-promoter DNA methylation (panel a) is the opposite from the global pattern (panel b,Supplementary Fig. S8). This suggestsHNF1BDNA methylation is not a passenger event of global DNA-methylation changes. Figure 2: HNF1B -promoter DNA methylation, protein expression and global DNA-methylation pattern by subtype. Each row is a tissue sample collected at the Mayo Clinic that belongs to one of the three categories: normal ovarian tissue ( n =7), clear cell ovarian tumours ( n =17) or serous ovarian tumours ( n =196). Endometrioid ( n =49) and mucinous ( n =7) tumours are not included in this figure. Each column represents a CpG locus, either from the region flanking the HNF1B transcription start site (panel A, ordered by genomic locations with an arrow indicating the transcription start site) or from a global panel of 1,003 CpG loci mapped to autosomal CpG island regions that distinguish clear cell and serous subtypes (panel B, ordered by average DNA methylation across the samples). For each horizontal panel group, the samples (rows) are ordered by HNF1B IHC status. The heatmap shows the DNA-methylation beta value, with blue indicating low DNA methylation and red indicating high methylation. Clear cell tumours showed less DNA methylation at the HNF1B -promoter region and correspondingly higher HNF1B protein expression. The clear cell tumours generally show a CIMP where there is extensive gain of aberrant promoter methylation in a correlated manner. CIMP status (left side bar, defined as methylated at >80% of the 1,003 loci) is highly correlated HNF1B expression. Also noteworthy is that the HNF1B -promoter DNA methylation (panel a) is the opposite from the global pattern (panel b, Supplementary Fig. S8 ). This suggests HNF1B DNA methylation is not a passenger event of global DNA-methylation changes. Full size image Although most clear cell tumours were devoid of HNF1B -promoter methylation, they revealed a surprisingly high frequency of CpG island hypermethylation at other sites across the genome, indicative of a CpG island methylator phenotype (CIMP). The few clear cell tumours lacking HNF1B expression exhibited HNF1B -promoter methylation, and a correspondingly low frequency of CpG island methylation throughout the genome, similar to the serous subtype ( Fig. 2 ). HNF1B expression and CIMP methylation are strongly associated ( P =3 × 10 −16 ; Fig. 2 ). Further, minimal hypermethylation is observed in serous tumours overall, but HNF1B is one notable exception ( Supplementary Fig. S7 ). DNA methylation and genotype We further investigated the relationship between risk allele genotypes and HNF1B DNA methylation in 231 serous ovarian cancers. The top serous risk SNP, rs7405776, showed only a borderline association with increased promoter methylation ( P =0.07; Fig. 3 ). Intriguingly, the association between SNPs in HNF1B and HNF1B -promoter DNA methylation strengthened as their location approached the promoter region, and the strongest signal came from a few SNPs, exemplified by rs11658063, overlapping with a polycomb repressive complex 2 (PRC2) mark in embryonic stem cells ( P =0.003; Fig. 3 , Supplementary Fig. S8 ). We validated this SNP–methylation association in the TCGA data ( Supplementary Fig. S9 ; see Methods ). None of the probes used contained common SNPs in the sequence, excluding technical artifact as a confounder of this association. 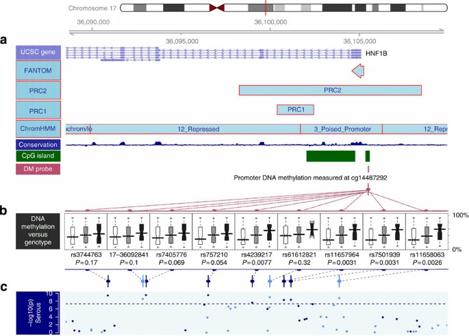Figure 3: Correlation of serous risk-associated SNPs withHNF1B-promoter DNA-methylation level. Plotted is the linkage disequilibrium region defined asr2>0.2 with the top serous SNP rs7405776. (a) Annotation of the region in terms of (from top to bottom:) UCSC genes, FANTOM mark, PRC marks (PRC2 and PRC1)32, the chromatin status determined in stem cells33, the conservation score across this region and the CpG island information, on top of the location of the HM450 probe used inbboxplots of promoter DNA-methylation level ofHNF1B(cg14487292) by SNP genotype with position indicated inc. This DNA-methylation probe was selected based on inverse association with mRNA expression forHNF1B, and does not contain any SNP with MAF >1% in its probe sequence. Each boxplot shows the distribution of DNA-methylation level by genotype (homozygous major—white; heterozygous—grey; and homozygous minor—black, where the minor alleles are the risk alleles). Two-sidedP-values testing for trend are presented, and are computed for 231 Mayo Clinic high-grade, high-stage serous tumours to avoid confounding by histological subtypes, and also to be consistent with the TCGA data (primarily high-grade, high-stage serous). Results were similar with all subtypes combined. The risk alleles are associated with significantly increased DNA methylation. The association of rs11658063 genotype with promoter methylation is consistent across the entire region flankingHNF1Btranscription start site, and stronger for the upstream promoter region (Supplementary Fig. S8). Figure 3: Correlation of serous risk-associated SNPs with HNF1B -promoter DNA-methylation level. Plotted is the linkage disequilibrium region defined as r 2 >0.2 with the top serous SNP rs7405776. ( a ) Annotation of the region in terms of (from top to bottom:) UCSC genes, FANTOM mark, PRC marks (PRC2 and PRC1) [32] , the chromatin status determined in stem cells [33] , the conservation score across this region and the CpG island information, on top of the location of the HM450 probe used in b boxplots of promoter DNA-methylation level of HNF1B (cg14487292) by SNP genotype with position indicated in c . This DNA-methylation probe was selected based on inverse association with mRNA expression for HNF1B , and does not contain any SNP with MAF >1% in its probe sequence. Each boxplot shows the distribution of DNA-methylation level by genotype (homozygous major—white; heterozygous—grey; and homozygous minor—black, where the minor alleles are the risk alleles). Two-sided P -values testing for trend are presented, and are computed for 231 Mayo Clinic high-grade, high-stage serous tumours to avoid confounding by histological subtypes, and also to be consistent with the TCGA data (primarily high-grade, high-stage serous). Results were similar with all subtypes combined. The risk alleles are associated with significantly increased DNA methylation. The association of rs11658063 genotype with promoter methylation is consistent across the entire region flanking HNF1B transcription start site, and stronger for the upstream promoter region ( Supplementary Fig. S8 ). Full size image Overexpression of HNF1B Given the proposed role of HNF1B in clear cell tumorigenesis, we stably overexpressed the gene in immortalized endometriosis epithelial cells (EECs), which are hypothesized to be a cell of origin for clear cell ovarian cancers ( Supplementary Fig. S10 ) [18] . EECs overexpressing HNF1B acquired an enlarged, flattened morphology and multi-nucleated cells accumulated in the cultures ( Fig. 4a ). Also, significant upregulation of HNF1B-associated genes SPP1, DPP4, and ACE2 was observed upon HNF1B overexpression in EECs ( Fig. 4b ). 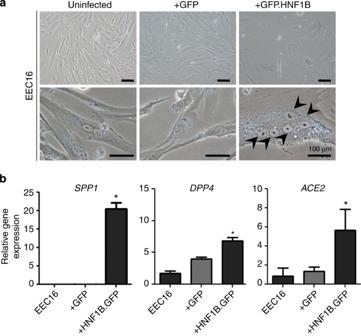Figure 4: Phenotypic effects and downstream targets of HNF1B overexpression in immortalized EECs. (a) Morphological changes in EECs expressing a HNF1B GFP fusion protein (EECGFP.HNF1B). GFP-positive cells were sorted using flow cytometry. The arrows indicate five nuclei contained within a single EECGFP.HNF1Bcell, showing the aberrant polynucleation that we observed in these cells. Using flow cytometry, we quantified the increase in polynucleation in EECGFP.HNF1Bto be around eightfold compared with controls (data not shown). (b) Gene-expression analysis ofHNF1B-target genes and clear cell ovarian cancer associated genes. *P>0.01. Figure 4: Phenotypic effects and downstream targets of HNF1B overexpression in immortalized EECs. ( a ) Morphological changes in EECs expressing a HNF1B GFP fusion protein (EEC GFP.HNF1B ). GFP-positive cells were sorted using flow cytometry. The arrows indicate five nuclei contained within a single EEC GFP.HNF1B cell, showing the aberrant polynucleation that we observed in these cells. Using flow cytometry, we quantified the increase in polynucleation in EEC GFP.HNF1B to be around eightfold compared with controls (data not shown). ( b ) Gene-expression analysis of HNF1B -target genes and clear cell ovarian cancer associated genes. * P >0.01. Full size image HNF1B appears to have a prominent role in ovarian cancer aetiology. It is the first clear cell ovarian cancer-susceptibility gene identified, and variation in the gene is also associated with risk of serous ovarian cancer at a genome-wide significance level. The gene is overexpressed in clear cell tumours and silenced in serous tumours. The strong association between HNF1B expression and CIMP methylation ( P =3 × 10 −16 ), and the reciprocal nature of DNA methylation at the HNF1B -promoter CpG islands, versus other CpG islands across the genome, suggests that HNF1B -promoter methylation is not merely a CIMP passenger event; in fact, HNF1B expression may even contribute to the hypermethylation phenotype. Taken together, these data indicate differing roles for HNF1B in these invasive EOC subtypes: a potential gain-of-function in clear cell ovarian cancer and loss-of-function in serous ovarian cancer, underscoring the heterogeneity of this disease. Different SNPs in the HNF1B gene regions explain the associations observed for serous and clear cell ovarian cancers. These different effects provide further support for the growing view that the histological subtypes of ovarian cancer represent distinct diseases [18] , [19] , [20] , [21] , [22] , [23] , [24] , with endometriosis as a proposed cell of origin for clear cell disease [18] and fallopian tube fimbriae as one for serous disease [22] . Interestingly, no association was observed between HNF1B genotypes and endometrioid ovarian cancer despite the view that, like clear cell, endometriosis is also a cell of origin for this subtype. The lack of association may be due to a different transformation mechanism from endometriosis for the endometrioid subtype, given that although the HNF1B promoter remains unmethylated in the endometrioid subtype, the endometrioid subtype does not overexpress HNF1B. Alternatively, misclassification of high-grade serous EOC as high-grade endometrioid could result in a bias towards the null for the endometrioid subtype. Variation in the 5′ UTR through the intron 4 region of HNF1B is also associated with susceptibility to prostate [12] , [14] , [15] , [16] and uterine cancer [17] (where minor alleles of certain SNPs are associated with decreased risk) and type II diabetes [12] , [13] (increased risk for the same or correlated SNP alleles; Supplementary Fig. S4 ). The opposing directions of these associations mirror the differential effects seen here in ovarian cancer. The most strongly associated SNP for both prostate [14] and uterine cancer [17] is rs4430796, correlated at r 2 =0.94 with the top clear cell ovarian cancer SNP, rs11651755, suggesting a common risk variant. Although increased risk of type II diabetes has been reported with rs4430796 (ref. 12 ), Winckler et al . [13] have suggested that the best marker of diabetes risk is rs757210, which correlated at r 2 =0.97 with our top serous SNP. Thus, the evidence suggests that a specific variant in HNF1B predisposes to clear cell ovarian, uterine and prostate cancers and that a different variants is associated with diabetes and serous ovarian cancer. We were able to completely fine-map the HNF1B region, localize the signal and identify a handful of potentially causal SNPs. This is quite different from other regions of the genome where it is not uncommon to identify hundreds of candidate causal SNPs. Further, an important link, often missing when susceptibility loci are identified, is the functional role that the variant has in disease. In the case of serous ovarian cancer, the SNP– HNF1B -promoter DNA methylation association strengthens as it approaches the promoter region, particularly where it overlaps with a PRC2 mark. PRC2–DNA methyltransferase cross-talk has been proposed to be a mechanism of predisposition to cancer-specific hypermethylation [25] . Our DNA-methylation data indicate that the causal risk alleles for the serous subtype may predispose the promoter to acquiring aberrant methylation, thereby promoting the development of serous but not clear cell tumours. This predisposition could be a direct functional effect of the SNP on the DNA-methylation machinery, or could act indirectly through differential binding affinity for PRC2 or one or more transcription factors. Given that we were able to fine-map the HNF1B region, it is unlikely that an unidentified common variant explains these associations. For serous ovarian cancer, the methylation signal suggests that the causal variant is most likely to be among those located within the region with the PRC2 mark for which we identified five SNPs with genome-wide significance. This is the first study investigating the effects of overexpression of HNF1B in endometriosis, and the results support the hypothesis that HNF1B may have an oncogenic role in the initiation of clear cell ovarian cancers, as speculated by Gounaris et al . [23] as a key step of endometriosis transformation. The observation in our data that HNF1B induces a polynucleated phenotype in EEC cells is intriguing, as clear cell ovarian cancers are often tetradiploid, more so than other ovarian cancer subtypes [26] . The polynucleated phenotype may suggest that HNF1B overexpression in EECs perturbs cytokinesis, causing aneuploidy in some cells. Histology re-review of the three clear cell tumours that do not express HNF1B revealed two scenarios: two samples with inconsistent evaluations between pathologists, and one consistently called clear cell. They might be cases that are especially difficult to classify, and therefore a molecular signature, for example, CIMP or HNF1B status, would be of great help in correctly classifying those tumours. The one sample that is called consistently clear cell tumour but does not express HNF1B might represent a rare subtype of clear cell carcinoma. With a larger cohort of clear cell ovarian cancers, these possibilities can be investigated. To our knowledge, this is the first report of tumour DNA-methylation patterns leading to the identification of a germline susceptibility locus, underscoring the value of TCGA. Recent studies suggest a strong genetic component to inter-individual variation in tumour DNA methylation, and demonstrate both cis- and trans - associations between genotypes and DNA methylation [27] . In addition, methylation quantitative trait loci were found to be enriched for expression quantitative trait loci. It has also been shown that epimutation is associated with genetic variation, for example, associations have been demonstrated between 5′ UTR MLH1 variants and MLH1 epigenetic silencing [28] . Moreover, we have for the first time demonstrated the existence of a CIMP phenotype in ovarian cancer, highlighting the complicated nature of the disease. In summary, variation in HNF1B is associated with serous and clear cell subtypes of ovarian cancer in opposite manner at genetic, epigenetic and protein expression levels. These observations are compatible with a tumour suppressor role in serous cancer and an oncogenic role in clear cell disease. Future efforts should focus on understanding these mechanisms as they could have major clinical implications for ovarian cancer, based on better subtype stratification, potential novel treatment approaches and a better understanding of disease aetiology. Currently, effective chemotherapeutics for clear cell ovarian cancer is lacking, but our study reveals that HNF1B-expressing clear cell tumours have extensive epigenetic alterations that potentially make them good candidates for epigenetic therapies. Molecular aspects TCGA data access We downloaded the TCGA serous ovarian cancer data packages from the TCGA public-access ftp ( https://tcga-data.nci.nih.gov/tcgafiles/ftp_auth/distro_ftpusers/anonymous/tumour/ov/ ). Data generated with the following platforms were used: Affymetrix HT Human Genome U133 Array Plate Set; Agilent 244K Custom Gene Expression G4502A-07-3; Affymetrix Human Exon 1.0 ST Array; and Illumina Infinium HumanMethylation27 Beadchip (a full list of the packages is provided in Supplementary Methods ).The Illumina Human1M-Duo DNA Analysis BeadChip Genotype data were downloaded from the controlled access data tier. DNA methylation data production for the OCRF tumour panel The Illumina Infinium HumanMethylation27 assay was performed as described [9] on 32 serous and 4 clear cell ovarian tumours from USC Norris Comprehensive Cancer Center and Duke University (‘OCRF tumour panel’). The beta values for each sample and locus were calculated with mean non-background corrected methylated (M) and unmethylated (U) signal intensities with the formula M/(M+U), representing the percentage of methylated alleles. Detection P -values were calculated by comparing the set of analytical probe replicates for each locus to the set of 16 negative control probes. Data points with detection P -values >0.05 were masked. DNA methylation data production for the Mayo tumour panel We also performed the Infinium HumanMethylation450 BeadChip assay on an independent set of tumour DNA in the Mayo Clinic Genotyping Shared Facility using recommended Illumina protocol [29] . 1 μg of tumour DNA was bisulfite-converted using the Zymo EZ96 DNA Methylation Kit. Three samples failing quality control were removed, leaving DNA-methylation data on 333 ovarian cancer cases, including 254 serous and 17 clear cell tumours. Plate normalization was done with a linear model on the logit-transformed beta values, following back-transformation to the (0,1) range. IHC assay Previously built tissue microarrays, triplicate core, measuring 0.6 mm were cut at 4-μm thickness and mounted on superfrost slides. Slides were stained on a Ventana Benchmark XT using the manufacturer’s pretreatment protocol CC1 standard ( Supplementary Methods ). A pathologist (MK) evaluated the IHC staining, and assigned the sample a score 0 in the absence of any nuclear staining, score 1 for any nuclear staining >1–50% or score 2 for >50% tumour cell nuclei-positive for HNF1B. Genotype and DNA methylation association We assessed the correlation of germline genotype at the nine genome-wide significant SNPs in serous cancer, with HNF1B DNA promoter methylation status using the Mayo Tumour Panel. Probe cg14487292 was used as it was most inversely correlated with mRNA expression. The nominal P -values are from two-sided tests for linear trend in the DNA-methylation beta values across the three genotypes for each locus. Bonferroni adjustment was not done for multiple comparisons as the SNPs are highly correlated. Validation was done with the TCGA data ( Supplementary Appendix ). In vitro model of HNF1B overexpression An immortalized EEC line was generated by lentiviral transduction of hTERT (Addgene plasmid 12245) into primary EECs ( Supplementary Fig. S10 ). TERT- immortalized EECs were transduced with lentiviral HNF1B-green fluorescent protein (GFP) or GFP (Genecopoeia) supernatants and positive cells selected with 400 ng ml −1 puromycin (Sigma). GFP expression was confirmed by fluorescent microscopy; HNF1B expression was confirmed by real-time PCR ( Supplementary Fig. S10 ). For gene-expression studies, RNA was collected from cells using the Qiagen RNeasy kit with on-column DNase I digestion. An amount of 1 μg RNA was reverse transcribed using an MMLV reverse transcriptase enzyme (Promega), and relative mRNA level was assayed using the ABI 7900HT Fast Real-Time PCR system utilizing the delta-delta Ct method. Statistical analyses were performed using Prism. Two-tailed paired t -tests with significance level of 0.05 were used. Genetic association study Study design The genetic susceptibility aspect of this study was organized by the Collaborative Oncological Gene-Environment Study, an ovarian, breast and prostate cancer consortium. The ovarian cancer part of this effort on which the current report is based is led by the Ovarian Cancer Association Consortium and included 43 studies ( Supplementary Table S1 ). Following sample quality control, 44,308 subjects, including 16,111 patients with invasive EOC, 2,063 with low malignant potential (borderline) disease and 26,134 controls, were available for analysis; results presented here are restricted to invasive cancers. All studies obtained approval from their respective human research ethics committees, and all participants provided written informed consent. Selection of SNPs Data for 174 SNPs in this region were available from the Collaborative Oncological Gene-Environment Study genotyping effort and provided full fine-mapping information in the 150-kb region surrounding HNF1B (hg18 coordinates 33,100,000–33,250,000). In addition, phase I haplotype data from the 1000 Genomes Project (January 2012) were used to impute genotypes for SNPs across this region, resulting in available data on an additional 307 SNPs with MAF >0.02 in European Whites and imputation r 2 >0.30 (IMPUTE 2.2). SNP genotyping The Ovarian Cancer Association Consortium genotyping was conducted by McGill University and Génome Québec Innovation Centre ( n =19,806) and the Mayo Clinic Medical Genome Facility ( n =27,824) using an Illumina Infinium iSelect BeadChip. Genotypes were called using GenCall. Sample and SNP quality-control measures are described in the Supplementary Methods . Statistical analysis We used the program LAMP [30] for principal components analysis to assign intercontinental ancestry based on the HapMap (release no. 22) genotype frequency data for European, African and Asian populations ( Supplementary Methods ). For LAMP-derived European ancestry groups for all patients of invasive cancer and for those with serous invasive cancer, we carried out unconditional logistic regression analyses within each study site, adjusted for the first five eigenvalues from the principal components analysis for European ancestry and then used a fixed-effects meta-analytic approach to obtain the summary OR estimate, 95% confidence interval and P -value. Details on analysis for the non-European groups are provided in the Supplementary Methods . Log-additive mode of inheritance was modelled (that is, co-dominant), treating each SNP as an ordinal variable. For haplotype analysis, we used the tagSNPs program [31] to obtain the haplotype dosage for each subject for the LAMP-derived European ancestry group for haplotypes with a frequency of ≥1%. The associations between haplotype and risks of serous and clear cell ovarian cancer were modelled by meta-analysis relative to the most common haplotype. How to cite this article: Shen, H., Fridley, B. L., Song, H. et al . Epigenetic analysis leads to identification of HNF1B as a subtype-specific susceptibility gene for ovarian cancer. Nat. Commun. 4:1628 doi: 10.1038/ncomms2629 (2013).